The rice mitochondrial iron transporter is essential for plant growth In plants, iron (Fe) is essential for mitochondrial electron transport, heme, and Fe-Sulphur (Fe-S) cluster synthesis; however, plant mitochondrial Fe transporters have not been identified. Here we show, identify and characterize the rice mitochondrial Fe transporter (MIT). Based on a transfer DNA library screen, we identified a rice line showing symptoms of Fe deficiency while accumulating high shoot levels of Fe. Homozygous knockout of MIT in this line resulted in a lethal phenotype. MIT localized to the mitochondria and complemented the growth of Δ mrs3 Δ mrs4 yeast defective in mitochondrial Fe transport. The growth of MIT -knockdown ( mit-2 ) plants was also significantly impaired despite abundant Fe accumulation. Further, the decrease in the activity of the mitochondrial and cytosolic Fe-S enzyme, aconitase, indicated that Fe-S cluster synthesis is affected in mit-2 plants. These results indicate that MIT is a mitochondrial Fe transporter essential for rice growth and development. Like other organisms, plants require iron (Fe) to complete their life cycle. Fe is essential for several cellular processes, such as respiration, chlorophyll biosynthesis and photosynthetic electron transport [1] . Fe exists in multiple redox states, readily accepting and donating electrons, permitting it to serve as a cofactor for several proteins such as components of the electron transport chain in mitochondria and chloroplast. In mitochondria, Fe is essential for the synthesis of heme by ferrochelatase [2] , and for the synthesis of Fe–sulphur cluster-containing proteins (Fe-S proteins) of both the matrix (for example, aconitase and homoaconitate hydratase) and the inner membrane [3] , [4] . Thus, limiting the supply of Fe to mitochondria impairs the metabolic and respiratory activities of this organelle and also affects Fe-S proteins in the cytoplasm [5] . On the other hand, excess Fe is toxic through the generation of reactive oxygen species. Free Fe ions might be particularly harmful to mitochondria, where free reactive oxygen species are generated as a side reaction of electron transport. In yeast, the alteration of mitochondrial activity by the inhibition of mitochondrial Fe transport leads to Fe accumulation in vacuoles and Fe deficiency in the cytoplasm. Mrs3 and Mrs4 are yeast ( Saccharomyces cerevisiae ) mitochondrial solute carrier family proteins transporting Fe into mitochondria under conditions of low-Fe availability [6] , [7] . MRS3-MRS4 knockout yeast (Δ mrs3 Δ mrs4 ) accumulates more Fe compared with wild-type (WT) strain and unable to grow well in Fe-limiting medium. The disturbance in mitochondrial Fe transport may result in high Fe accumulation in cytoplasm. To avoid this, the activity of yeast vacuolar Fe transporter Ccc1 increases resulting in increased Fe accumulation in vacuole and rendering the cytoplasm Fe deficient [8] . As a result, the Fe uptake system is triggered ultimately accumulating more Fe [7] . Although Fe is abundant in soils, it is not easily available, as it is mainly present as oxidized compounds which are poorly soluble in neutral to alkaline soils. Thus the uptake, translocation and storage/recycling of Fe is extremely important for normal growth of plants. Plants have developed sophisticated mechanisms to acquire Fe from soil [9] . Graminaceous plants use a chelation strategy to acquire Fe from soil and secrete mugineic acid family phytosiderophores. Furthermore, rice is capable of absorbing Fe as Fe(II) [10] as well as Fe(III)-deoxymugineic acid (DMA). The biosynthetic pathway of mugineic acid (MA) has been studied in detail and all the genes involved in the biosynthesis of DMA have been cloned [11] . In addition, transporters involved in the absorption and translocation of Fe in rice have been characterized. OsYSL15 (ref. 12 ) and OsIRT (ref. 10 ) were reported to be Fe(III)-DMA and Fe(II) transporters, respectively, which take up Fe from the rhizosphere. OsYSL2 is an Fe(II)-nicotianamine and manganese (Mn) (II)-nicotianamine transporter responsible for the phloem transport of Fe and Mn [13] . Arabidopsis acquires Fe from rhizosphere through IRT [14] . Vacuolar Fe transporter (AtVIT1 (ref. 15 )) and PIC1, the chloroplast Fe transporter, have also been characterized [16] . Additionally, several proteins involved in Fe homeostasis in plants have been characterized [17] , [18] . Despite the rapid progress in understanding Fe uptake and homeostasis, the protein transporting Fe into the mitochondria has not been identified in plants. Here we report the cloning and characterization of a m itochondrial i ron- t ransporter ( MIT ) gene in rice. Our results suggest that MIT is essential for plant growth and development. The cloning of MIT is an important advancement in understanding plant-cellular-Fe transport and for developing strategies to mitigate wide spread Fe deficiency problem. Screening T-DNA library and identification of MIT We screened a rice transfer DNA (T-DNA) library consisting of 3,993 independent lines for symptoms of Fe deficiency (that is, chlorotic new leaves and green old leaves) to identify genes with a significant role in Fe transport. This criterion was set to avoid the identification of plants defective in chlorophyll biosynthesis and/or related defects. We identified a line harbouring a T-DNA insertion in the second exon of Os03g0296800 (later named mitochondrial Fe transporter, MIT ; Fig. 1a,b ). The respective T-DNA insertion line ( mit-1 ) was analysed; however, we failed to find any plants homozygous for this knockout. Growth of the mit-1 heterozygous plants was also significantly affected ( Fig. 1c ), although they accumulated 2.5 times more shoot Fe than WT plants, when grown in soil ( Fig. 1d ). We analysed individual seeds collected from mit-1 heterozygous plants to examine the segregation of homozygous and heterozygous plants in the progeny. Surprisingly, only 7 and 23% of the seeds were homozygous and heterozygous for T-DNA integration, compared with the expected segregation ratio of 25 and 50%, respectively ( Fig. 1e ). After germination, no homozygous seedling was identified, and the ratio of heterozygous seedlings also dropped ( Fig. 1e ). 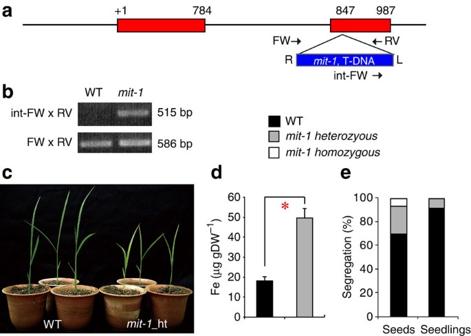Figure 1: Screening of a T-DNA library and identification ofmit-1plants. (a) Genomic organization ofMITand T-DNA integration inmit-1plants. Red boxes represent exons. (b) Confirmation of heterozygous status ofmit-1plants. The position of primers is shown in (a), FW, forward; RV, reverse are located on genomic DNA; int-FW, internal forward for T-DNA. (c) Phenotype ofmit-1heterozygous plants. (d) Fe concentration ofmit-1heterozygous plants; μg per /gDW−1: μg/gram dry weight. (e) Segregation analysis ofmit-1heterozygous plants usingmit-1seeds (n=27) and seedlings (n=32). The graph shows mean±s.d.; *P<0.05, ANOVA followed by a Student-Newman-Keuls test,n=3. Figure 1: Screening of a T-DNA library and identification of mit-1 plants. ( a ) Genomic organization of MIT and T-DNA integration in mit-1 plants. Red boxes represent exons. ( b ) Confirmation of heterozygous status of mit-1 plants. The position of primers is shown in ( a ), FW, forward; RV, reverse are located on genomic DNA; int-FW, internal forward for T-DNA. ( c ) Phenotype of mit-1 heterozygous plants. ( d ) Fe concentration of mit-1 heterozygous plants; μg per /gDW−1: μg/gram dry weight. ( e ) Segregation analysis of mit-1 heterozygous plants using mit-1 seeds ( n =27) and seedlings ( n =32). The graph shows mean±s.d. ; * P <0.05, ANOVA followed by a Student-Newman-Keuls test, n =3. Full size image MIT localizes to mitochondria and complements the growth of Δ mrs3 Δ mrs4 A homology search ( http://www.blast.ncbi.nlm.nih.gov/Blast.cgi ) confirmed the presence of the conserved regions of mitochondrial solute carrier family (MSC) proteins in MIT (amino acids from 134–166 and 171–223). MIT-green fluorescent protein (GFP) localized to mitochondria, when expressed in tobacco BY-2 cells whereas GFP alone, used as control, localized to the cytoplasm ( Fig. 2a–f ). 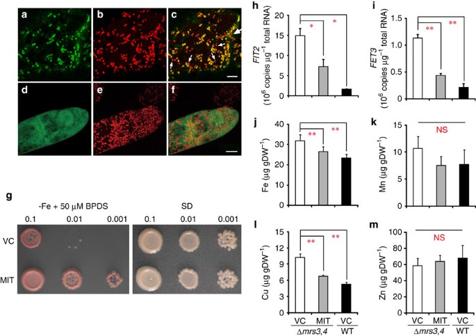Figure 2: Subcellular localization and yeast complementation assay of MIT. (a–f). MIT-GFP expression in suspension cultured tobacco BY2 cells. (a,d): GFP fluorescence; (b,e): MitoTracker red fluorescence; (c,f): merged image. (a–c): MIT∷sGFP; (d–f): sGFP. Scale,a–c, 5 μM,d–f, 10 μM. (g) Representative of serial dilutions of Δmrs3Δmrs4cells transformed with MIT or empty vector placed onto control SD medium or SD medium with 50 μM BPDS (n=6). (j–m): Metal concentration of Δmrs3Δmrs4and WT yeast transformed with MIT or VC; μg g DW−1: μg per gram dry weight. The graph shows mean±s.d.; *P<0.05, **P<0.001; NS, not significant; ANOVA followed by a Student-Newman-Keuls test,n=3. BPDS, batho-phenanthroline disulfonic acid; SD, synthetic defined medium; VC, vector control/empty vector. Figure 2: Subcellular localization and yeast complementation assay of MIT. ( a – f ). MIT-GFP expression in suspension cultured tobacco BY2 cells. ( a , d ): GFP fluorescence; ( b , e ): MitoTracker red fluorescence; ( c , f ): merged image. ( a – c ): MIT ∷ sGFP; ( d – f ): sGFP. Scale, a – c , 5 μM, d – f , 10 μM. ( g ) Representative of serial dilutions of Δ mrs3 Δ mrs4 cells transformed with MIT or empty vector placed onto control SD medium or SD medium with 50 μM BPDS ( n =6). ( j – m ): Metal concentration of Δ mrs3 Δ mrs4 and WT yeast transformed with MIT or VC; μg g DW −1 : μg per gram dry weight. The graph shows mean±s.d. ; * P <0.05, ** P <0.001; NS, not significant; ANOVA followed by a Student-Newman-Keuls test, n =3. BPDS, batho-phenanthroline disulfonic acid; SD, synthetic defined medium; VC, vector control/empty vector. Full size image MIT expressed in Δ mrs3 Δ mrs4 yeast mutants complemented the growth defect of the mutant yeast ( Fig. 2g ). In Δ mrs3 Δ mrs4 yeast, the expression of Fe uptake genes is upregulated [7] . The upregulation of FIT2 and FET3 is reverted to wild-type levels upon expression of the rice gene ( Fig. 2h,i ). Moreover, it also reversed the changes in accumulation of Fe and Cu ( Fig. 2j–m ). These results suggested a clear role for MIT in Fe homeostasis. Expression pattern of MIT in rice Quantitative RT–PCR revealed that the transcripts of MIT were three times lower in the roots and shoots of plants exposed to Fe-limited conditions compared with plants grown hydroponically in the presence of 100 μM Fe. MIT transcripts were increased in the roots and shoots when the plants were exposed to excess Fe (500 μM Fe; Fig. 3a,b ). To further understand its role during germination and seed development, the MIT promoter was used to drive the expression of β- glucuronidase in rice. MIT expression was observed during germination and at all stages of seed development. During germination, MIT expression was specific to the embryo ( Fig. 3c–f ). Expression was observed in the leaf primordia and coleorhizae 1 day after germination ( Fig. 3d ). It increased subsequently and, 3 days after germination, was observed in whole embryo ( Fig. 3f ). Expression was also observed from anthesis through seed development ( Fig. 3g , left to right), supporting the hypothesis that MIT has a crucial role in these growth stages. Further the steady state transcripts of MIT were observed during all growth stages of rice plant including root, leaves, stem, anther, pistil, lemma, palea, ovary, embryo and endosperm as revealed by microarray analysis ( Supplementary Fig. S1 ). 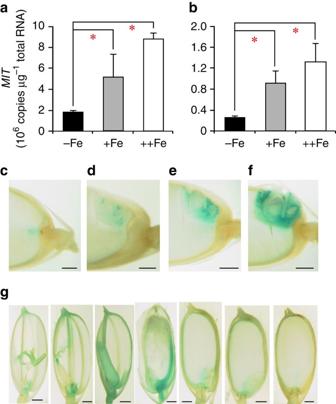Figure 3: Expression analysis ofMIT. (a,b) The changes in expression ofMITin response to Fe availability −Fe: 0 μM Fe; +Fe: 100 μM Fe; ++Fe: 500 μM Fe. (a) Root. (b) Shoot. (c–g)MITpromoter driven β-glucuronidaseexpression during germination (c–f) and seed development (g); (c) 0; (d) 1; (e) 2; (f) 3 days after germination. (g) From left to right, before anthesis 1, 4, 12, 16, 20 and 25 days after anthesis. Scale, 500 μm. The graph shows mean±s.d.; *P<0.05, ANOVA,n=3. Figure 3: Expression analysis of MIT . ( a , b ) The changes in expression of MIT in response to Fe availability −Fe: 0 μM Fe; +Fe: 100 μM Fe; ++Fe: 500 μM Fe. ( a ) Root. ( b ) Shoot. ( c – g ) MIT promoter driven β- glucuronidase expression during germination ( c – f ) and seed development ( g ); ( c ) 0; ( d ) 1; ( e ) 2; ( f ) 3 days after germination. ( g ) From left to right, before anthesis 1, 4, 12, 16, 20 and 25 days after anthesis. Scale, 500 μm. The graph shows mean±s.d. ; * P <0.05, ANOVA, n =3. Full size image Characterizing the MIT knock down mutant As the homozygous knockout of MIT in mit-1 plants proved lethal, we characterized MIT -knockdown ( mit-2 ) plants ( Fig. 4 ). Hydroponically grown mit-2 plants were smaller than similarly grown WT plants ( Fig. 4a ; Supplementary Fig. S2 ). PCR analysis confirmed the integration of the T-DNA 604 bp upstream of the start codon and the homozygous status of mit-2 plants ( Supplementary Fig. S2a,b ). Moreover, quantitative RT-PCR analysis confirmed that the expression of MIT in the mit-2 plants was reduced compared with WT plants ( Fig. 4b ). There was a significant reduction in root and shoot dry weight as well as in the root and shoot length, leaf width and chlorophyll content ( Supplementary Fig. S2c–h ). Hydroponically grown mit-2 plants accumulated 51% more Fe than WT plants in the shoots ( Fig. 4c ). The accumulation of Mn was also changed ( Fig. 4d ) whereas no change in the accumulation of Cu and Zinc (Zn) was observed ( Supplementary Fig. S2i,j ). 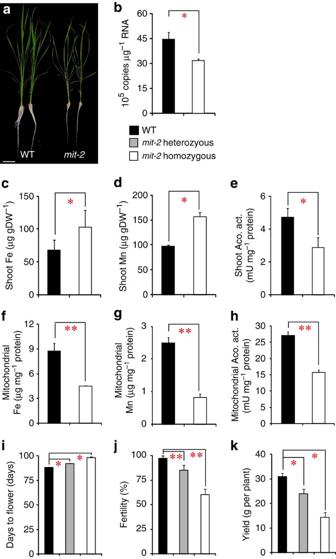Figure 4: Characterization ofmit-2plants. (a). Phenotype of hydroponically grown WT andmit-2plants. Scale, 10 cm. (b)MITexpression inmit-2shoots. (c,d). Fe and Mn contents of WT andmit-2shoots; μg g DW−1: μg per gram dry weight. (e). Total aconitase activity of WT andmit-2shoots; 1 mU: n mol min−1per mg protein). (f,g). Fe and Mn contents of WT andmit-2isolated mitochondria. (h). Mitochondrial aconitase activity. (i–k) Morphological characteristics of soil grown WT andmit-2plants. The graph shows mean±s.d.; *P<0.05, **P<0.001; ANOVA followed by a student-Newman-Keuls test,n=3. Figure 4: Characterization of mit-2 plants. ( a ). Phenotype of hydroponically grown WT and mit-2 plants. Scale, 10 cm. ( b ) MIT expression in mit-2 shoots. ( c , d ). Fe and Mn contents of WT and mit-2 shoots; μg g DW −1 : μg per gram dry weight. ( e ). Total aconitase activity of WT and mit-2 shoots; 1 mU: n mol min −1 per mg protein). ( f , g ). Fe and Mn contents of WT and mit-2 isolated mitochondria. ( h ). Mitochondrial aconitase activity. ( i – k ) Morphological characteristics of soil grown WT and mit-2 plants. The graph shows mean±s.d. ; * P <0.05, ** P <0.001; ANOVA followed by a student-Newman-Keuls test, n =3. Full size image Mitochondria isolated from shoot tissue of mit-2 plants accumulated less Fe compared with WT mitochondria. Mitochondrial Fe concentration of mit-2 plants was 49% less, compared with mitochondria isolated from WT plants ( Fig. 4f ). Changes in Mn and Cu accumulation were also observed ( Fig. 4g ; Supplementary Fig. S2k ). The expression of aconitase genes was not changed in mit-2 plants ( Table 1 ), whereas the total and mitochondrial aconitase activity decreased in the mit-2 plants compared with WT plants. In shoot tissue, the total aconitase activity of mit-2 was 39% less compared with WT plants, whereas a reduction of 42% was observed for the mit-2 aconitase activity from isolated mitochondria ( Fig. 4e,h ). Table 1 Summary of microarray analysis of MIT knockdown plants ( mit-2 ). Full size table The growth of the mit-2 plants in soil was also significantly impaired compared withWT plants. The average number of tillers in the mit-2 plants was 8 compared with 20 in the WT plants; in addition, the mutants were compromised in terms of plant height ( Supplementary Fig. S2m,n ). Flowering was delayed in the mit-2 plants, and fertility was also significantly lower, reducing the yield by 59% compared with that in WT plants ( Fig. 4i–k ). Although the growth of soil-grown mit-2 heterozygous plants was impaired compared with that of WT plants, it was superior to that of mit-2 homozygous plants for all these characteristics ( Fig. 4i–k ;& Supplementary Fig. S2m,n ), confirming that the phenotype was specific to the mit-2 plants. As mitochondrial activity is important for cell division, we generated calli from WT and mit-2 plants; the size and weight of the calli was significantly reduced in the mit-2 calli compared with the WT ( Supplementary Fig. S2o ). Complementing mit-2 with MITp-MIT To determine whether the mit-2 phenotype is specifically caused by the reduced expression of MIT , mit-2 plants were transformed with MIT open reading frame (ORF) governed by the MIT promoter. As the mit-2 plants were previously transformed with T-DNA and were selected on hygromycin, second transformation was done using rice ALS gene [19] as selection marker. The expression of MIT in mit-2 plants significantly reversed the growth defect in terms of plant height, chlorophyll content as well as Fe and Mn accumulation ( Fig. 5 ). 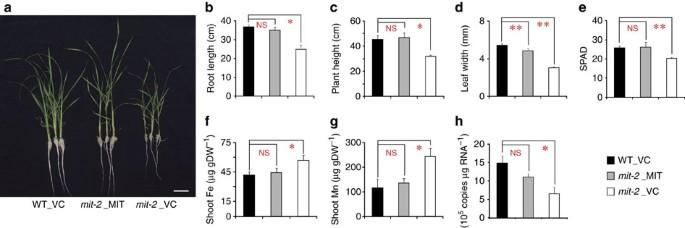Figure 5: Characterization ofmit-2plants complemented with MITp-MIT. (a–d) Morphological characteristics of hydroponically grown WT plants transformed with empty vector (WT_VC) andmit-2plants transformed with MIT ORF (mit-2_MIT) or empty vector (mit-2_VC). (a) Phenotype of hydroponically grown plants. Scale, 10 cm. (b) Root length. (c) Shoot length. (d) Leaf width. (e–g) Fe and Mn content of hydroponically grown plants. (h) Expression of MIT in hydroponically grown plants. The graph shows mean±s.d.; *P<0.05, **P<0.001; NS, not significant; ANOVA followed by a student-Newman-Keuls test, WT andmit-2plants;n=3,mit-2-MITplants;n=5. Figure 5: Characterization of mit-2 plants complemented with MITp-MIT. ( a – d ) Morphological characteristics of hydroponically grown WT plants transformed with empty vector (WT_VC) and mit-2 plants transformed with MIT ORF ( mit-2 _MIT) or empty vector ( mit-2 _VC). ( a ) Phenotype of hydroponically grown plants. Scale, 10 cm. ( b ) Root length. ( c ) Shoot length. ( d ) Leaf width. ( e – g ) Fe and Mn content of hydroponically grown plants. ( h ) Expression of MIT in hydroponically grown plants. The graph shows mean±s.d. ; * P <0.05, ** P <0.001; NS, not significant; ANOVA followed by a student-Newman-Keuls test, WT and mit-2 plants; n =3, mit-2-MIT plants; n =5. Full size image Microarray analysis Microarray analysis of mit-2 plants was performed to determine whether the change in MIT expression affected other Fe homeostasis-related genes in rice plants. Our results indicate that MIT expression was significantly reduced in the mit-2 plants ( Table 1 ). Moreover, the expression of a homologue of the Arabidopsis vacuolar Fe and Mn transporter [15] ( OsVIT1 ), homologue of Arabidopsis Fe efflux transporter [20] ( OsFerroportin ) was significantly upregulated in the mit-2 plants, and the expression of ferritin, an Fe storage protein [21] , was also slightly upregulated. On the other hand, expression of the genes upregulated by Fe deficiency was downregulated; for example, expression of the Fe(II) transporters OsIRT1 , OsIRT2 (ref. 6 ) and Fe(III)-DMA transporter OsYSL15 (ref. 12 ) was slightly downregulated in the roots. Similarly, the expression of rice ferric chelate reductase OsFRO2 (ref. 10 ) was decreased in the shoots, whereas expression of the Fe transporter OsNramp1 (ref. 22 ), and Fe(II)-nicotianamine transporter OsYSL2 (ref. 13 ) was downregulated in the roots. Like other eukaryotes, plant mitochondria depend much on Fe for normal function; however, the proteins transporting cytoplasmic Fe across the mitochondrial membrane have not been characterized. We screened a rice T-DNA mutant library and identified a plant showing Fe-deficiency symptoms when grown under Fe-sufficient conditions, accumulating higher Fe compared with WT plants, and resulting in a lethal phenotype. Further studies revealed that T-DNA is integrated in to a gene encoding MIT. MIT knock out mutation caused a growth defect during seed development as revealed by the analysis of mit-1 heterozygous plants examined for the segregation of homozygous and heterozygous plants in the progeny. These analyses further revealed that, although to a lesser extent, MIT also has a role in germination. Besides producing a lethal phenotype for knockout mutant, the knockdown mutation also resulted in a severe phenotype and the growth of mit-2 was also significantly impaired when grown hydroponically, or in soil. Although growth was also impaired in mit-2 heterozygous plants compared with WT plants, soil grown mit-2 heterozygous plants were superior to mit-2 homozygous plants for agronomical characteristics such as average number of tillers, fertility and yield. The heterozygous plants were also superior to mit-2 homozygous plants in terms of plant height and days to flowering confirming that the mit-2 phenotype is specific to MIT knockdown plants. Both mit-1 heterozygous and mit-2 homozygous plants accumulated higher Fe in shoot tissue compared with WT plants. The impaired growth, despite the higher accumulation of Fe, indicated that plants may not be able to utilize the accumulated Fe. Metal profiling of mitochondria isolated from shoot tissue of mit-2 plants was significantly different from WT for Fe accumulation, whereas changes in Mn and Cu accumulation were also observed. Thus, in mit-2 plants, reduced MIT expression leads to low Fe transport to mitochondria, leaving the cytoplasm with slightly elevated Fe levels. Changes in mitochondrial Fe accumulation could affect the Fe-S cluster synthesis in mitochondria. In line with this, the total and mitochondrial aconitase activity decreased in the mit-2 plants compared with WT plants, showing that Fe-S cluster synthesis was significantly affected in mit-2 plants. The reduction in the chlorophyll soil-plant analysis development (SPAD) value may be due to problems in mitochondrial Fe-S cluster synthesis that indirectly affect the chloroplasts. It has already been shown that knockout plants for the mitochondrial-synthesized Fe-S cluster exporter exhibit chlorosis [23] . The lethal phenotype of mit-1 plants and the significantly impaired growth of the mit-2 plants, complementation of mit-2 plants with MIT and phenotype of mit-2 heterozygotes highlight the importance of MIT in plant growth and development. On the other hand, the Fe-related phenotype and reduced aconitase activity in mit-2 plants indicate that MIT is essential for Fe homeostasis in rice. A complete loss of MIT may be lethal, whereas a reduction in MIT expression (as in mit-1 heterozygous and mit-2 plants) significantly affects mitochondrial activity. This reduced activity may affect several cellular functions, which force the plant to compromise on important agronomic parameters. MIT belongs to the MSC family of proteins. The members of this family localize to the inner mitochondrial membrane, have conserved regions and transport a wide range of substrates, including Fe [24] , [25] . The MSC family members transporting Fe into the mitochondria have been characterized in several organisms including yeast (Mrs3-Mrs4 (ref. 7 )), mouse [26] , Drosophila [27] and zebrafish [28] (mitoferrin). The mitoferrin has been characterized in detail and the interactions of ferrochelatase, mitoferrin-1 and Abcb10 has also been revealed [29] . MIT has 39, 41 and 42% homology to Mrs3, Mrs4 and mitoferrin, respectively; whereas phylogenetic analysis revealed the absence of any close homologue in rice ( Supplementary Fig. S3 ). The yeast Δ mrs3 Δ mrs4 phenotype is only significant under low-Fe conditions (in the presence of Fe a substantial amount of Fe is imported into mitochondria), indicating that it is not the only MIT, although it is the only high-affinity MIT in yeast [30] . Besides Fe, Mrs3–Mrs4 also transport copper (Cu) [31] . In the yeast Δ mrs3 Δ mrs4 double mutant, activity of the yeast vacuolar Fe and Mn transporter Ccc1 increases to avoid Fe toxicity in the cytoplasm, resulting in increased Fe and Mn accumulation in the vacuole and Fe deficiency in the cytoplasm [7] , [8] . As a result, the Fe-uptake system is triggered leading to a greater accumulation of these metals in the cells compared with the WT strain. MIT localized to mitochondria and complemented the growth defect of Δ mrs3 Δ mrs4 yeast mutants confirming that MIT has the same function as Mrs3p/Mrs4p. The expression of MIT in yeast reversed the upregulation of FIT2 and FET3 found in the Δ mrs3 Δ mrs4 mutant and also reversed the changes in accumulation of Fe, and Cu. These results also suggested a clear role of MIT in cellular Fe homeostasis. The mutation in rice MIT is lethal, as Fe participates in vital processes in the mitochondria, including the electron transport chain and the synthesis of haem and Fe-S proteins [2] , [3] , [4] . Zebrafish expressing a mutant version of mitoferrin had severely hypochromic erythrocytes [28] , whereas Arabidopsis defective in frataxin which is involved in Fe-S cluster assembly, had a lethal phenotype [32] . Mutation in rice specific mitochondrial iron-regulated gene also resulted in severe phenotype [17] . The transcripts of MIT increased in the roots and shoots when the plants were exposed to excess Fe (500 μM Fe), and decreased under Fe-limiting conditions, indicating that the steady state MIT transcript levels are regulated by iron. Further expression of MIT was observed during germination, through vegetative stage in roots and leaves, and during seed development to support the hypothesis that MIT has a crucial role in these growth stages. Microarray analysis of mit-2 plants revealed significant changes in the expression of genes regulated by Fe. The mit-2 plants accumulated more Fe than the WT plants, thus, it is not surprising that genes related to Fe sequestration were upregulated and expression of genes involved in Fe uptake decreased. In yeast Δ mrs3 Δ mrs4 , the expression of genes regulated by Fe deficiency as well as Ccc1 is upregulated. It appears that rice uses a different strategy compared with yeast to tackle the reduced expression of MIT ( Supplementary Fig. S4 ). This difference may be explained by the fact that higher plants need more complex control of Fe homeostasis compared with yeast, a unicellular eukaryote. In brief, through library screening, we cloned a major MIT essential for plant growth and development. Reduced MIT expression affected mitochondrial activity, including Fe-S cluster synthesis, and impaired plant growth and development, especially at the reproductive stage. As rice is a staple food for a large portion of the human population, understanding Fe homeostasis and improving the Fe content of rice are major objectives for rice researchers [33] to mitigate widespread Fe deficiency in humans. The characterization of MIT is a significant step in advancing these efforts. Identification and characterization of the mutant lines Approximately 30,000 seeds, from 3,993 independent lines of a rice T-DNA library of japonica cultivar Dongjing transformed with p2715 (ref. 34 ) were grown hydroponically and screened for the presence of mutants showing symptoms of Fe deficiency. Three plants were selected, and iPCR was performed, as described in ref. 35 to identify the point of T-DNA integration. Finally, one plant was identified that harboured the T-DNA in the second exon of Os03g0296800 . Further, the respective T-DNA line ( mit-1 ) was analysed for integration of the T-DNA by PCR using a T-DNA-specific primer (5′-AATATCTGCATCGGCGAACTGATCG-3′), and an mit-1 -specific FW primer (5′-GCTGTCATTGAGTTGTGCAC-3′) and mit-1 -specific RV primer (5′-TGAATGTTCAGATTATTTCC-3′). This line was further analysed for the presence of homozygous mit-1 plants, and seed DNA extracted from 27 independent seeds were analysed with the following primers: T-DNA internal forward (5′-CTCGTATGTTGTGTGGAATTGTGA-3′) and T-DNA internal reverse (5′-GTAGAACGGTTTGAGGTTAATCAGGAAC-3′), and with primers specific for the borders of the T-DNA integration site (forward [5′-GCTGTCATTGAGTTGTGCAC-3′] and reverse [5′-GAACAGCATTCTTGGCTTCC-3′]). T-DNA integration in the mit-2 plants was confirmed using the T-DNA-specific primer 5′-AATATCTGCATCGGCGAACTGATCG-3′ and mit2 -specific RV primer 5′-GTAGGGTTAGGGTTTAGACGC-3′. To confirm the homozygous status of the mit-2 , primers located near the T-DNA integration site, mit-2 -specific FW (5′-CCAACTTGGTCACTAGATCTGG-3′ and mit-2 -specific RV were used as forward and reverse primers, respectively. Similarly, the seeds were germinated on tissue paper and analysed 1 day after germination for segregation. Subcellular localization of MIT The full-length ORF of MIT was amplified with forward and reverse primers (5′-caccATGGCCGCCGACTACCGCACACC-3′ and 5′-TTATTTCCTTCTTTTCTCGTTGA-3′, respectively), subcloned into pENTR/D-TOPO (Invitrogen), and sequenced. The MIT ORF was then subcloned into pH7WGF2 (ref. 36 ). Tobacco BY-2 cells were transformed, and the expression of GFP was observed as described previously [37] . Complementation of Δ mrs3 Δ mrs4 mutant yeast Δ mrs3 Δ mrs4 mutant yeast and the respective WT strain (BY4741) [7] were transformed with empty vector (pHY23) or vector containing the MIT ORF. The yeast strains were grown on synthetic defined (SD) medium as described [7] . For complementation assays, agarose was used instead of agar to avoid Fe contamination. Yeast strains were grown in liquid SD medium, and serial dilutions were prepared (OD 600 ) as 0.1, 0.01 and 0.001 and plated onto SD plates. The plates were incubated at 30 °C for 6 days. RNA was extracted using Qiagen RNeasy total RNA extraction kit (QIAGEN). For quantitative RT-PCR, following primers were used: FIT2 forward, 5′-GACACCGCTGACCCTA TCAT-3′, and reverse as 5′-AGGCAGAAGAGGAGGAGGAG-3′, FET3 forward 5′-ACGGTGTGAATTACGCCTTC-3′, and reverse as 5′-TGGAAAGCGTGACCATGTAA-3′. For normalizing data, the following UBC6 specific primers were used: forward 5′-GATACTTGGAATCCTGGCTGGTCTGTCTC-3′, and reverse as 5′-AAAGGGTCTTCTGTTTCATCACCTGTATTTGC-3′. Rice transformation and growth conditions The 1.7-kb 5′-flanking region of MIT was amplified by PCR using genomic DNA as template with the forward primer 5′-CACCCTATCTTTCAAGCTTGGAGCTTGCCTTTTCG-3′ and reverse primer 5′-CGGCGGCCATTCTAGAGGAGGGCGGCTGCGGTAGG-3′, which contain a Hin dIII restriction site. The amplified fragment was fused into the pBluescript II SK+ vector, and its sequence confirmed. The MIT promoter was digested with Xho I and Bgl II, and the digested 1.7-kb fragment was subcloned upstream of the uid A ORF, which encodes β-glucuronidase, in the pIG121Hm vector [38] . Oryza sativa L. cv. Tsukinohikari was transformed by using the agrobacterium-mediated transformation method. The plants were grown in a greenhouse; the histochemical localization of MIT was observed in three independent T2 plants as described [10] . Characterization of the mutants mit-1 and mit-2 plants were either grown hydroponically or in soil. The morphological characters like plant height, average number of tillers, days to flower and fertility percentage were recorded as described [39] . An aconitase assay was performed using an aconitase assay kit (Biovision) as suggested by the manufacturer. For measuring metal concentration in WT and mutants, Leaf or root samples were digested with 3 ml of 13 M HNO 3 at 220 °C for 20 min using a MARS XPRESS microwave reaction (CEM) in triplicate. After digestion, samples were collected and diluted to 5 ml and elemental analysis of the WT, mit-1 and mit-2 plants were performed using inductively coupled plasma atomic emission spectrometry (SPS1200VR; Seiko) as described [40] . Mitochondria were isolated from WT and mit-2 plants grown hydroponically for three weeks as described [41] . Briefly, shoot tissue from 120 WT and mit-2 plants, grown hydroponically for 3 weeks, were grinded in the presence of buffer (450 mM Sucrose, 1.5 mM EGTA, 15 mM MOPS, pH 7.4, 0.2% BSA, 0.6% PVP, 10 mM DTT and 0.2 mM PMSF), purified through three layers of mira cloth, centrifuged at 3,500 g twice (first time 10 min and second time 5 min); the supernatant was centrifuged at 6,000 g for 5 min and mitochondria were pelleted by centrifugation at 17,000 g for 10 min. The pellet was dissolved in buffer containing 300 mM sucrose, 1 mM EGTA, 10 mM MOPS, pH 7.2 and loaded on to a Percoll gradient and centrifuged for 45 min at 70,000 g and mitochondria were recovered between 29% and 45% percoll. All the steps were performed at 4 °C. For microarray analysis, seeds of the mit-2 plants were germinated on Murashige and Skoog (MS) medium and transferred to hydroponic solution 10 days after germination and grown for three weeks in the presence of 100 μM Fe. Roots and shoots were collected, frozen in liquid nitrogen, and stored at −80 °C until use. RNA was extracted from the roots and shoots of three plants, and total RNA (200 ng) from the mit-2 , and WT plants were labelled with Cy3 or Cy5 using an Agilent Low RNA Input Fluorescent Linear Amplification Kit (Agilent Technologies), and microarray analysis was performed in duplicate, according to the manufacturer's instructions, using a rice 44 K oligo-DNA microarray (Agilent). The data has been deposited in GEO under the accession number GSE28428 . Points with a P -value <0.001, and a ratio >2 in both the Cy3 and Cy5 channels, were considered to be significantly upregulated. The data regarding expression of MIT was generated through Rice global gene expression profile data sets [42] ( http://www.ricexpro.dna.affrc.go.jp/index.html ). Quantitative RT-PCR for MIT was performed with the forward and reverse primers 5′-CAAGACTCAGCTGCAGTGTC-3′ and 5′-GAACAGCATTCTTG GCTTCCA-3′, respectively, as described [43] . The primers used for internal control in RT-PCR were α -tubulin forward, (5′-TCTTCCACCCTGAGCAGCTC-3′) and α -tubulin reverse (5′-AACCTTGGAGACCAGTGCAG-3′). Complementation of mit-2 with MIT For complementation analysis, MIT ORF was subcloned into pR-5 (Kumiai Chemicals), and the 1.7 kb promoter region was subcloned with Xba 1 and Hin dIII restriction sites. As the mit-2 plants contain T-DNA and were selected on hygromycin, for complementation analysis, plants were transformed using Oryza sativa W548L/S627I ALS gene [19] and sodium 2,6-bis(4,6-dimethoxypyrimidin-2-yloxy) benzoate as selection marker. WT plants transformed with empty vector and mit-2 plants with either empty vector, or pR5 containing MITp-MIT were grown hydroponically for two weeks and metal profiling and morphological analysis were performed. Statistical analysis To determine whether the observed differences between the WT and mit plants were statistically significant, one-way ANOVA was performed using Costat 6.400 (Cohort, USA) with a completely randomized design followed by a Student-Newman-Keuls test ( P <0.05). Accession codes: The microarray data have been deposited in Gene Expression Omnibus database under the accession codes GSE28428 . How to cite this article: Bashir, K. et al . The rice mitochondrial iron transporter is essential for plant growth. Nat. Commun. 2:322 doi: 10.1038/ncomms1326 (2011).